Multiple reentrant glass transitions in confined hard-sphere glasses Glass-forming liquids exhibit a rich phenomenology upon confinement. This is often related to the effects arising from wall–fluid interactions. Here we focus on the interesting limit where the separation of the confining walls becomes of the order of a few particle diameters. For a moderately polydisperse, densely packed hard-sphere fluid confined between two smooth hard walls, we show via event-driven molecular dynamics simulations the emergence of a multiple reentrant glass transition scenario upon a variation of the wall separation. Using thermodynamic relations, this reentrant phenomenon is shown to persist also under constant chemical potential. This allows straightforward experimental investigation and opens the way to a variety of applications in micro- and nanotechnology, where channel dimensions are comparable to the size of the contained particles. The results are in line with theoretical predictions obtained by a combination of density functional theory and the mode-coupling theory of the glass transition. A thorough understanding of the slowing down of transport by orders of magnitude upon approaching the glass transition is one of the grand challenges of condensed matter theory [1] , [2] , [3] , [4] , [5] . A recent focus in the study of glasses has been to introduce competing mechanisms that lead to glass transition phase diagrams exhibiting non-monotonic behaviour. Reentrant scenarios have been uncovered, for example, upon adding a short-range attraction to colloidal particles [6] , [7] , [8] , by competing near ordering in binary mixtures [9] , [10] , or by inserting the liquid in a frozen disordered host structure [11] , [12] , [13] . However, instead of changing the structure of the liquid directly, one may also affect its properties by purely geometric means, via an increase of its confinement [14] , [15] , [16] , [17] , [18] , [19] , [20] , [21] , [22] , [23] , [24] . Depending on the ratio of the characteristic confinement length (for example, the wall separation) to particle diameter, this can either lead to an increase or decrease of the first peak of the pair distribution function—the latter being a measure of the ‘stiffness’ of the local packing structure [18] . As long as crystallization is kinetically hindered, this is expected to have a strong impact on the dynamics of the liquid and the glass transition. Earlier simulation studies and experiments of the confinement effects on the glass transition were mainly concerned with wall-to-wall separations of the order of several particle diameters or larger (see, for example, refs 14 , 15 , 16 , 17 , 18 , 19 and references therein). Recently, however, the case of stronger confinement has received growing attention [20] , [21] , [22] , [23] . Here we focus on this latter regime of strong confinement, where only a few particle layers fit into the space between the walls. The problem of crystallization is circumvented by introducing size dispersity [25] into our simulations, which leads to a geometric frustration. We evaluate the diffusion coefficient to assess the slowing-down of the dynamics and to establish a glass-transition state diagram. Typical snapshots from our molecular dynamics (MD) simulations are shown in Fig. 1 , where the colouring indicates the particle diffusivity and serves to visualize the non-monotonic effects on the dynamics due to confinement. A drastic enhancement of confinement effects on the system’s dynamics is observed as the packing fraction approaches the glass transition. We transfer our results to the experimentally easily accessible situation of a wedge-shaped channel filled with colloidal hard-sphere particles and provide evidence for the coexistence of alternating liquid-glass regions along the wedge. These findings for the simulated polydisperse hard-sphere system are corroborated by theoretical calculations based on a combination of density functional–integral equation theory and mode-coupling theory (MCT) of the glass transition [26] for monodisperse confined hard-sphere liquids [21] , [27] , [28] . 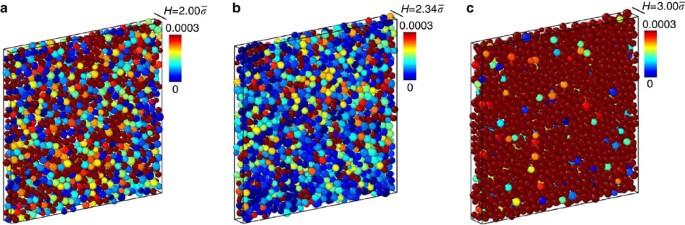Figure 1: Diffusivity of individual particles. Snapshots of the simulation box for three selected plate separations of(a),(b) and(c). The packing fraction isϕ=0.50 in all the three cases shown. The colour encodes the diffusivity of individual particles, defined viaDi≡limt→∞‹[xi(t)−xi(0)]2›/2t, where in practicetis chosen sufficiently large to reflect diffusive motion. The system is periodic in the directions parallel to the walls. In all the three cases shown, the colour scale indicates the diffusion coefficient. It ranges from (in hard-sphere units)D=0 (blue) toD=0.0003 (brown). Figure 1: Diffusivity of individual particles. Snapshots of the simulation box for three selected plate separations of ( a ), ( b ) and ( c ). The packing fraction is ϕ =0.50 in all the three cases shown. The colour encodes the diffusivity of individual particles, defined via D i ≡lim t →∞ ‹[ x i ( t )− x i (0)] 2 ›/2 t , where in practice t is chosen sufficiently large to reflect diffusive motion. The system is periodic in the directions parallel to the walls. In all the three cases shown, the colour scale indicates the diffusion coefficient. It ranges from (in hard-sphere units) D =0 (blue) to D =0.0003 (brown). Full size image Static properties The strong confinement induces structural changes of the liquid because of competing length scales. Layering effects become manifest in an oscillatory density profile along the direction perpendicular to the wall, n ( z ), see Fig. 2 . The simulations clearly display accumulation of particles close to the walls, z =± H /2, and upon increasing the plate distance more oscillations emerge. The theoretical n ( z ) for monodisperse hard spheres shares the same oscillatory structure, although the peaks at the walls are here located at the contact distances and are more pronounced. The difference to the simulations is due to the polydispersity as we have checked by explicit calculations using fundamental-measure theory (FMT; Supplementary Fig. 1 ). 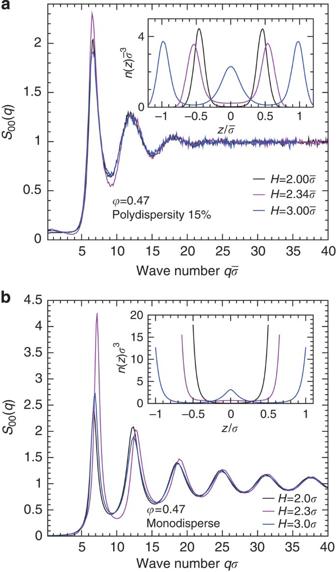Figure 2: Structure and density due to confinement. (a) Simulated static structure factorS00(q) for different plate distancesHat packing fractionϕ=0.47. The first sharp diffraction peak varies non-monotonically; lowest forand, highest for. Inset: the density profiles for various wall-to-wall distances at the same packing fraction. (b) Structure factor forϕ=0.47 obtained from Percus–Yevick theory with density profilesn(z) as obtained from fundamental-measure theory. Figure 2: Structure and density due to confinement. ( a ) Simulated static structure factor S 00 ( q ) for different plate distances H at packing fraction ϕ =0.47. The first sharp diffraction peak varies non-monotonically; lowest for and , highest for . Inset: the density profiles for various wall-to-wall distances at the same packing fraction. ( b ) Structure factor for ϕ =0.47 obtained from Percus–Yevick theory with density profiles n ( z ) as obtained from fundamental-measure theory. Full size image The structure factor S 00 ( q ) ( q being the wavevector parallel to the walls) is similar in overall shape to bulk liquids. Simulations reveal already at this level a non-monotonic variation manifested in a steep shoot-up of the first sharp diffraction peak for non-commensurate wall distances. For the distances investigated, the maximum appears for , where is the average particle diameter, see Fig. 2 . Within the Percus–Yevick approximation for monodisperse hard spheres, the maximum of the peak occurs at the same wall separation, however, the peaks are more pronounced and the oscillations persist to larger wave numbers. The structural features in the simulations are smeared because of polydispersity. This is evidenced in Supplementary Fig. 2 , where a decrease of polydispersity is shown to enhance the non-monotonic effect of confinement on S 00 ( q ). The quality of the Percus–Yevick closure has been corroborated recently for confined systems [29] . The qualitative agreement between the theory for monodisperse confined hard spheres and the simulation for hard spheres with size dispersity on the static level is a prerequisite to compare computer simulation and MCT for the dynamics in the vicinity of the glass transition. Empirical studies of the MCT solutions for several components in bulk [30] demonstrate only slight quantitative changes with respect to the monodisperse case and also the pioneering experiments [31] on hard spheres (4% polydispersity) have been quantitatively rationalized within the one-component MCT. It appears thus promising to compare also in this context the simulations of polydisperse hard spheres to the single-component MCT. Diffusivities and state diagram A first glimpse of the non-monotonic dependence of the dynamics on plate separation is illustrated in Fig. 1 , where particles are coloured according to their individual diffusivity with their initial position. Clearly, the intermediate wall separation has the largest number of slow particles (blue) compared with the other two cases shown ( and ). For a quantitative analysis, we have determined the film average mean-square displacement in the direction parallel to the walls for a wide range of plate separations and packing fractions. As evidenced in Fig. 3 , the dynamics of the confined system is significantly suppressed with respect to the bulk. Beginning at and increasing H at constant packing fraction, the dynamics first slows down and the characteristic plateau at a length scale of extends to longer times. Separating the walls even more, the dynamics becomes faster again, such that the plateau region almost disappears. Similar to the static structure, a reduction of polydispersity leads to an enhancement of this non-monotonic confinement effect ( Supplementary Fig. 3 ). 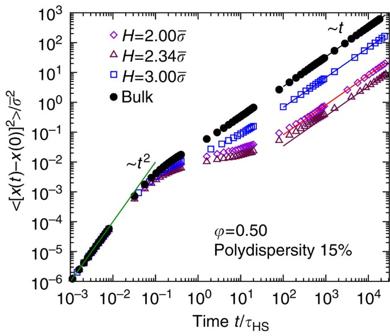Figure 3: Mean-square displacement for both bulk and confined systems. The film average mean-square displacement in the direction parallel to the walls for the same plate separations and packing fraction as inFig. 1. For reference, the bulk data of the same packing fraction are also shown. The polydispersity is 15% andτHSdenotes the microscopic time scale of the hard-sphere system (see Methods). Figure 3: Mean-square displacement for both bulk and confined systems. The film average mean-square displacement in the direction parallel to the walls for the same plate separations and packing fraction as in Fig. 1 . For reference, the bulk data of the same packing fraction are also shown. The polydispersity is 15% and τ HS denotes the microscopic time scale of the hard-sphere system (see Methods). Full size image We have investigated whether the confinement generates segregation effects for the polydisperse system, that is, a redistribution of particle sizes in zones close to and distant from the wall. Our results show no sign of wall-induced segregation ( Supplementary Fig. 4 ). Moreover, we have determined the pair-distribution function to check for the occurrence of confinement-induced long-range order; and we have only taken those ϕ - H -values into account for which the pair-distribution function exhibits a liquid-like structure ( Supplementary Fig. 5 ). We also observe that dynamic heterogeneity [32] strongly enhances as packing fraction increases ( Supplementary Note 1 and Supplementary Fig. 6 ). This provides further evidence for the glassy dynamics in the selected parameter range. The diffusion coefficient D of the hard-sphere fluid ( Fig. 4 ) is extracted as an average over all the particles in the system from the long-time behaviour of the mean-square displacement of the particles by D =lim t →∞ ‹[ x ( t )− x (0)] 2 ›/2 t ; a reliable criterion here to have reached the diffusive regime is that . The diffusion constant is measured in units of , where τ HS denotes the microscopic time scale of the hard-sphere system (see Methods). A non-monotonic dependence of D on the plate separation has been observed already for moderate densities [20] with modulations of about a factor of 2. As seen in Fig. 4 , increasing the packing fraction leads to a dramatic enhancement of confinement effects in the vicinity of the— H -dependent—glass transition. At ϕ =0.52 (15% polydispersity), for example, the diffusion coefficient varies by a factor of 1,000 upon a variation of H . This amplification in the densely packed regime is one of our principal results and could only be achieved by introducing polydispersity. The slightly shorter dynamic range in the case of 10% polydispersity is related to the onset of the above-mentioned wall-induced long range order for ϕ >0.49. The strong non-monotonic variation of the diffusion coefficient at fixed packing fraction upon changing the wall separation is a direct dynamic manifestation of commensurate and incommensurate packing effects arising from the inhomogeneous structure. This finding can be rationalized by comparing the diffusion coefficients for 10 and 15% polydispersity ( Fig. 4 ). Since the structure is less inhomogeneous for increasing polydispersity (compare left panel of Fig. 2 with Supplementary Fig. 2 ), this behaviour is directly reflected in less pronounced non-monotonic effects in the diffusion coefficient (compared, for example, in Fig. 4 for ϕ =0.49, the variations of D ( H ) for the two investigated polydispersities). 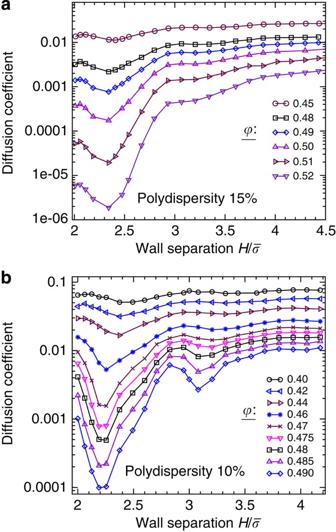Figure 4: Measurement of dynamical properties via diffusion coefficients. Diffusion coefficientDversus film thicknessHfor different packing fractionsϕfor two different polydispersities of (a) 15% and (b) 10%. The packing fraction increases from top to bottom. The confinement-induced oscillations become less pronounced as polydispersity decreases. Error bars are of the order of the symbol size. Figure 4: Measurement of dynamical properties via diffusion coefficients. Diffusion coefficient D versus film thickness H for different packing fractions ϕ for two different polydispersities of ( a ) 15% and ( b ) 10%. The packing fraction increases from top to bottom. The confinement-induced oscillations become less pronounced as polydispersity decreases. Error bars are of the order of the symbol size. Full size image The diffusivities remain monotonic as a function of the packing fraction ϕ for fixed wall distance. We have fitted a power law D ( ϕ ) ∝ ( ϕ c − ϕ ) γ to the data ( Fig. 5 ), which is asymptotically predicted by the (idealized) MCT [26] and persists under confinement [33] , [34] , [35] . We find that the exponent γ =2.1±0.1 is rather robust, and depends only weakly on polydispersity and H . Therefore, the fit probes essentially the critical packing fraction ϕ c . 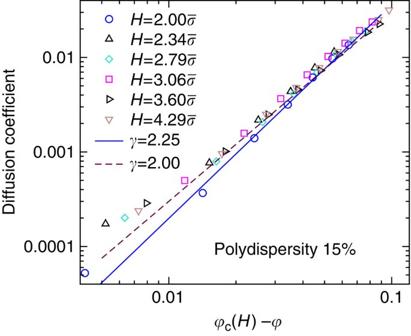Figure 5: Power-law fits for diffusion data. Idealized mode-coupling theory26fitsD(ϕ)∝(ϕc−ϕ)γ(straight lines) to the diffusion data obtained from simulations (symbols) for a polydispersity of 15%. Figure 5: Power-law fits for diffusion data. Idealized mode-coupling theory [26] fits D ( ϕ ) ∝ ( ϕ c − ϕ ) γ (straight lines) to the diffusion data obtained from simulations (symbols) for a polydispersity of 15%. Full size image We use the such extracted ϕ c ( H ) as an indicator for the glass-transition line. The state diagram relying on the extrapolated ϕ c ( H ) from the simulation is compared with the MCT calculations in Fig. 6 . The most prominent feature are oscillations with a period comparable to the hard-sphere diameter, emphasizing the competition of wall-induced layering and local packing. As a consequence, reentrant behaviour is generic on isopycnics (lines of constant density) upon gradually decreasing the wall distance. Along such paths (see arrows in Fig. 6b ), first a transition from a confined liquid to a non-ergodic glass state occurs, followed by a melting to a fluid state upon further shrinking the dimension. Contrary to reentrant phenomena induced by, for example, short-range attraction [7] , here the oscillations allow for multiple reentrants. 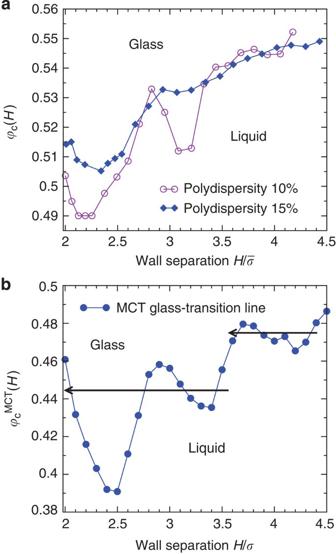Figure 6: Comparison of state diagram between simulation and theory. (a) State diagram of confined polydisperse hard spheres as obtained from power-law fits to our simulation results on the diffusion coefficient. (b) Numerical results from MCT for a confined hard-sphere fluid. The arrows indicate paths of equal densities where (multiple) reentrant behaviour occurs. Error bars are of the order of the symbol size. Figure 6: Comparison of state diagram between simulation and theory. ( a ) State diagram of confined polydisperse hard spheres as obtained from power-law fits to our simulation results on the diffusion coefficient. ( b ) Numerical results from MCT for a confined hard-sphere fluid. The arrows indicate paths of equal densities where (multiple) reentrant behaviour occurs. Error bars are of the order of the symbol size. Full size image The MCT calculations predict for 0.39≤ ϕ ≤0.46 another melting transition, which for ϕ =0.45 (see lower arrow in Fig. 6b ) is located at a plate separation of H =2.0 σ , and we anticipate a subsequent oscillation with a further minimum (similar to the coexistence lines of hard spheres at H = σ (refs 36 , 37 ) and joining the 2d limit, ϕ c ( H = σ ) ≅ 0.465, as predicted by the MCT for hard disks [38] . The simulation data for 10% polydispersity and the MCT result reveal an increase of the transition line at the lowest plate distances, corroborating this scenario. The enhanced oscillations at a lower polydispersity suggest the size dispersity to be an important cause for deviations between simulations and theory—the latter considering a perfectly monodisperse system ( Supplementary Note 2 ). Transferring results to a wedge-shaped confinement As isopycnic (constant density) experiments with a variable plate distance may be difficult to perform, we use thermodynamic relations (see Methods) to transfer the above results to the experimentally more accessible situation of a wedge-shaped geometry (see Fig. 7 ), which has been used in a similar context already [19] , [39] , [40] . For small tilt angle, θ , the plates are locally parallel and the fluid is in local thermal equilibrium, such that particle exchange along the wedge is possible. Hence, the chemical potential is constant throughout the system, whereas the channel width H = H ( x )= x tan( θ ) increases slowly along the wedge ( x is the distance from the corner, see Fig. 7 ). 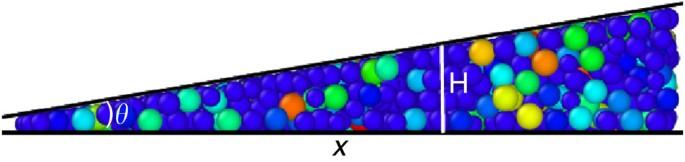Figure 7: Typical wedge. A snapshot of a polydisperse hard-sphere system in a wedge-shaped channel. The heightHobeysH=xtan(θ). Note that the tilt angleθ=9° here is much larger than in typical experiments. Figure 7: Typical wedge. A snapshot of a polydisperse hard-sphere system in a wedge-shaped channel. The height H obeys H = x tan( θ ). Note that the tilt angle θ =9° here is much larger than in typical experiments. 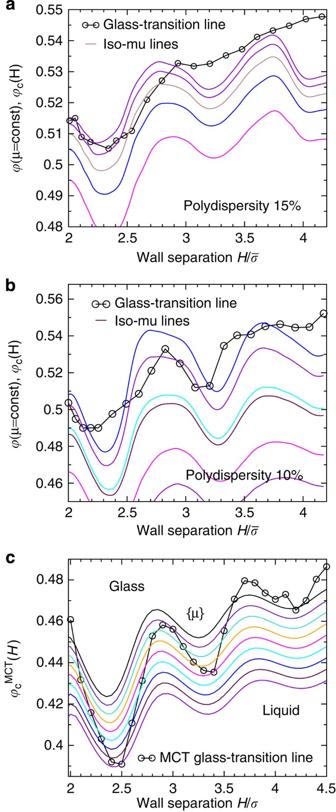Figure 8: Variation of density at constant chemical potential in a wedge. Lines of constant chemical potential (‘iso-μ lines’) as obtained from thermodynamic mapping of the simulated data at 10% (a) and 15% (b) polydispersity to the case of a wedge-shaped geometry. (c) The same quantity as obtained from fundamental-measure theory. Full size image Figure 8 shows the variation of density along the wedge channel for different values of the chemical potential (using the above given relation H = x tan( θ )). The existence of multiple crossing points between the glass-transition line and a line of constant chemical potential indicates that liquid and glass states can indeed coexist along a wedge. Figure 8: Variation of density at constant chemical potential in a wedge. Lines of constant chemical potential (‘iso-μ lines’) as obtained from thermodynamic mapping of the simulated data at 10% ( a ) and 15% ( b ) polydispersity to the case of a wedge-shaped geometry. ( c ) The same quantity as obtained from fundamental-measure theory. Full size image Direct simulations of the wedge at moderate packing fractions In order to provide further evidence for the non-monotonic scenario proposed in the present manuscript, we have also performed MD simulations of a polydisperse hard-sphere system in a wedge geometry with a tilt angle of θ =9°. These simulations demonstrate that the diffusion coefficient in a wedge exhibits oscillations as a function of the distance from the corner of the wedge ( Fig. 9 ). At a constant average packing fraction, these oscillations are most pronounced for the monodisperse system. In the case of a polydisperse system, similar effects are observed at higher average packing fractions, corresponding to higher chemical potentials or pressures. This strongly suggests that the anticipated liquid-glass phase-coexistence may indeed occur at a sufficiently high external pressure. We have performed a consistency check for the proposed transferal from parallel plates to a wedge. In Fig. 10 we display the packing fractions as a function of the wall separation obtained from direct simulations of the wedge and compare them to the density functional theory (DFT) calculations at constant chemical potential. Both simulation and theory show oscillations of the local packing fraction along the wedge and an enhancement of these oscillations upon increasing the average density (that is, total particle number) or chemical potential. The slight differences between simulation and theory probably stem from the finite tilt angle in the simulations and the related deviations from the assumption of locally parallel plates. 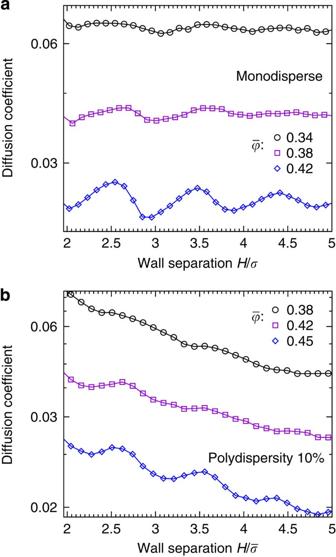Figure 9: Direct simulation results on the diffusion coefficient in a wedge versus local height H=xtan(θ). (a) A monodisperse system, (b) results for a polydispersity of 10%. The tilt angle isθ=9°.xrefers to the distance from the corner of the wedge. The average packing fractionis defined as the total volume occupied by all the particles divided by the volume of the wedge. Figure 9: Direct simulation results on the diffusion coefficient in a wedge versus local height H = x tan( θ ). ( a ) A monodisperse system, ( b ) results for a polydispersity of 10%. The tilt angle is θ =9°. x refers to the distance from the corner of the wedge. The average packing fraction is defined as the total volume occupied by all the particles divided by the volume of the wedge. 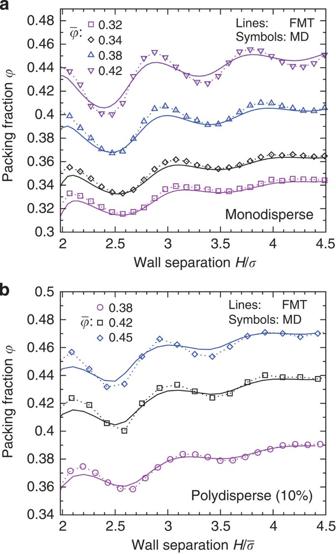Figure 10: Direct simulation results on packing fraction variation in a wedge. Symbols correspond to simulations, whereas solid lines are results of the DFT calculations at constant chemical potential. (a) A monodisperse system, (b) results for a polydispersity of 10%. The tilt angle isθ=9°. The average packing fractionis defined as the total volume occupied by all the particles divided by the volume of the wedge. Full size image Figure 10: Direct simulation results on packing fraction variation in a wedge. Symbols correspond to simulations, whereas solid lines are results of the DFT calculations at constant chemical potential. ( a ) A monodisperse system, ( b ) results for a polydispersity of 10%. The tilt angle is θ =9°. The average packing fraction is defined as the total volume occupied by all the particles divided by the volume of the wedge. Full size image Simulation results for the dynamics of a polydisperse hard-sphere fluid confined between two smooth hard walls reveal a dramatic change in the diffusion of hard spheres under confinement. In particular, glassy dynamics can be promoted or suppressed by varying the film thickness, whereas the packing fraction remains constant. The diffusion coefficient follows the idealized MCT prediction for all film thicknesses, supporting that MCT in confinement leads to the same universal scenario close to the glass-transition singularity as in the bulk, but with a H -dependent critical packing fraction. For not too strong polydispersity, also the resulting phase diagram is in qualitative agreement with the MCT prediction. We have shown for the first time the emergence of a multiple reentrant scenario for the case of a moderately polydisperse system in confined geometry. The interplay of several length scales is drastically enhanced near the glass-transition line. Our results reveal that the glass transition itself exhibits subtle incommensurability effects. These competing trends should manifest themselves also in the glass form factors as function of wavenumber and mode index. Similarly, the shape of the structural relaxation dynamics should contain valuable information on how commensurability controls the glass transition. The present study also sheds light onto the delicate role of polydispersity. Although on the one hand increasing size dispersity has a stabilizing effect on the metastable amorphous state, on the other hand it smears out the multiple-reentrant phenomenon. Our study thus suggests that, in order to keep this effect intact, the polydispersity must be selected with care. Finally, by transferring the present results to the case of a wedge-shaped channel, we predict that the reentrant effect also persists in this interesting, experimentally more accessible case. In such experiments, there would be no need to keep the density constant. Rather, by tuning the external pressure, it is possible to enforce the coexistence of alternating liquid-glass regions. The present findings motivate further investigations of confined hard-sphere glasses. Indeed, the glass transition is a rich field where small competing effects are enhanced drastically as manifested, for example, in the structural relaxation and diffusion. In this context, it would be interesting to investigate how the reentrant behaviour observed in this work affects other aspects of the glass transition, for example, cooperativity and dynamic heterogeneity [41] . A question of interest here is how, upon a variation of wall separation, the system approaches the quasi-2D behaviour corresponding to extreme confinement . Although for colloidal particles flat walls are easily implemented, for molecular liquids surfaces generically display some residual roughness on the Ångström scale. Computer simulations have revealed that the dynamics is slowed down, thereby shifting the glass transition lines to lower densities, while at the same time softening the layering within the structure [16] , [18] , [42] , [43] , [44] . Furthermore, we anticipate that studying densely packed binary mixtures in such narrow slits will exhibit additional intriguing phenomena. Binary mixtures already in bulk reveal interesting mixing effects as the composition and the size ratio of the constituents are changed [45] , [46] . The interplay with the confinement length scale suggests that, for a clever choice of the mixture, oscillations in the non-equilibrium state diagram in confinement could be significantly enhanced or, respectively, almost totally suppressed. Simulations We perform event-driven MD simulations of a polydisperse hard-sphere system in three dimensions [47] . The particle-size distribution is drawn from a Gaussian around a mean diameter of with two different polydispersities of 10 and 15%. The particles are confined between two planar hard walls placed in parallel at ± H /2 and periodic boundary conditions are applied along the lateral directions. The confined systems studied here cover the range of packing fractions ϕ from the normal liquid to the supercooled state, where a two-step relaxation with an extended plateau is clearly visible. Length is measured in units of the mean particle diameter , and time in terms of , where k B is the Boltzmann constant, T is temperature and m is the mass of a particle. We set m =1, k B =1 and T =1. The polydispersity is defined as the width of the Gaussian distribution function relative to the mean particle diameter. Here, the mean particle diameter serves as a ‘good’ measure as the distribution is narrow enough so that higher moments do not contain further information: . The centre of particle i with diameter σ i is confined to −( H −σ i )/2≤ z i ≤( H −σ i )/2. The volume of the simulation box is , where the lateral system size L box varies in the range from to . Depending on polydispersity, the packing fractions investigated lie in the range ϕ ε[0.4, 0.49] (10%) and ϕ ε[0.45 0.54] (15%). Depending on H , L box and ϕ , the number of particles ranges between 8,000 and 30,000. Thermal equilibrium is ensured by sufficiently long simulations (extending up to seven decades in time) and by explicitly testing the time-translation invariance of the properties of interest. Although large H and low ϕ is computationally inexpensive, significant effort is necessary in order to obtain accurate results for ( ϕ , H ) values with the slowest dynamics. For example, at 15% polydispersity, ten independent runs for ϕ =0.52 and are performed, each with a duration of roughly 6 weeks on a 3-GHz central processing unit (CPU). The structure of the liquid is characterized by the static structure factor S 00 ( q )= N −1 ‹ ρ 0 ( q )* ρ 0 ( q )›, ρ where is the particle density Fourier-transformed along the periodic direction, corresponding to particle coordinates r n =( x n , y n ) and wave vector q . The index ‘0’ signals the lowest order in a hierarchy of structure factors S μ ν ( q ) that include Fourier factors along the confined direction z as well. The matrix-valued character of the structure factor is a consequence of the broken translational and rotational symmetry of the confined system [21] , [27] , [28] . Theory We also employ MCT [26] to locate numerically the critical packing fraction ϕ c ( H ) of the liquid–glass transition as a function of the plate distance (wall-to-wall separation) H . MCT requires as input the static structure factors S μ v ( q ), obtained from integral equation theory for inhomogeneous fluids with the Percus–Yevick closure, and the density profile n ( z ), which we obtain here via density functional theory with fundamental-measure functionals [48] , [49] . Minimization of the functional for the grand free energy leads to the equation where n i ( z ) is the partial number density of component i (with diameter σ i ), μ i the chemical potential for component i, which is set by a particle reservoir, V i ( z ) is the wall potential (different for each component) and F ex is the excess free energy functional for a hard-sphere mixture from FMT (version White Bear II (ref. 49 ), currently the most precise and consistent hard-sphere mixture functional). We use n components to emulate polydispersity and have checked that n =11, 31, 51 yield indistinguishable results for the profile. We require that the bulk densities in the reservoir are taken from a Gaussian distribution as used in the simulation, and that the chemical potentials μ i correspond to these bulk densities. This results in partial species concentrations in the slit, which depend on the slit width and may deviate slightly from a Gaussian distribution. The theoretical result—obtained via FMT—shows qualitatively the same trend as in simulations ( Supplementary Fig. 1 ). The difference to the simulations is probably mainly due to the difference between slit and reservoir particle distributions. The same functional, but with n =1 (monodisperse hard spheres), has been used to calculate the slit density distribution n ( z ) necessary for obtaining the results of Fig. 2b and the iso-μ lines of Fig. 8c . As in density functional theory, the chemical potential μ is the external control parameter (see equation (1)), the iso-μ lines were obtained by simple scans of the μ - H parameter space where for each point ( μ , H ) the minimizing equation (1) has been solved. Using this microscopic approach, we have succeeded to generate structure factors for high densities, which allow us to calculate a glass-transition phase diagram from first principles. The linear approximation used in previous calculations [21] to estimate the transition has been overcome, thus providing accurate predictions for comparison with simulations or future experiments. We calculate the intermediate scattering function (ISF) characterizing the spatio-temporal dynamics. In bulk liquids, translational and rotational invariance imply that the ISF depends only on the magnitude of the wavevector. For confined systems, one has to generalize bulk MCT [21] , [27] , [28] to describe matrix-valued ISFs . Here, are symmetry-adapted Fourier modes for the microscopic density, where the first exponential factor accounts for the confinement along the z -direction with . The coordinate axes are chosen as ( x , y , z ), where lies in the plane parallel to the walls and z denotes the normal direction. The MCT has been derived only for single-component liquids; to make comparison with the polydisperse system, we associate the accessible width L of the slit with . Furthermore, we employ the static structure for an equivalent monodisperse confined hard-sphere liquid of diameter . Glass states are characterized by non-vanishing long-time limits of the ISF, F μ ν ( q )=lim t →∞ S μ ν ( q , t )≠0, referred to as glass form factors. The theory provides a closed set of equations to evaluate F μ ν ( q ), where the known static structure factors S μ ν ( q )= S μ ν ( q , t =0), as well as the average density profile n ( z ), enter as sole inputs. We have employed FMT [48] , [49] to evaluate n ( z ) and used a Percus–Yevick approximation to close the inhomogeneous Ornstein–Zernike relation [50] to solve for the structure factors. We have implemented the MCT fixed-point equation and have located numerically the critical packing fraction as a function of the plate distance H . In order to locate the location of the glass–liquid transition line for the distances H =2.0 σ , 2.1 σ ,…, 5.0 σ , the fixed point equation is solved by iteration to obtain . The discrete mode indices are truncated as | ν |≤10 and the wavevectors are discretized on a grid with parameters q 0 σ =0.1212 and Δ qσ =0.4, and grid range with N =75. To reduce computing time, only diagonal elements of matrix-valued quantities are included. These calculations are new and allow for the first time an accurate determination of the glass transition in the presence of confinement. In particular, the approach used here is free of the linearization approximation used in ref. 21 . Thermodynamic mapping to constant chemical potential Here we devise a simple procedure allowing to transfer the above results to the experimentally more accessible situation of variable channel width at constant chemical potential, rather than constant density. Such a situation may be realized, for example, in a wedge-shaped geometry. A liquid of N particles confined between two parallel flat walls of surface area A separated by a distance H (assumed to be comparable to the bulk correlation length) is characterized by a free energy F ( T , A , H , N ) ( T being the temperature). The free energy fulfills the fundamental thermodynamic relation where S is the entropy, μ is the chemical potential and p L and p N are the lateral and normal pressures, respectively. The extensivity of F implies that F ( T , A , H , N )= Nf ( T , a , H ), where f is the free energy per particle and a = A / N the area per particle. We thus obtain Comparing terms with equation (2) yields the fundamental relation for the free energy per particle with s ≡ S / N the entropy per particle, as well as the relations μ = f + ap L H and The thermodynamics of wedges has been studied extensively, mostly in the context of density functional theory [51] . Here we take a much simpler approach. For small tilt angles, the plates are almost parallel and the fluid can be viewed as being locally confined with a wall separation H . As particles are free to move along the wedge, each section is in chemical contact with its neighbours. Hence, the chemical potential along the wedge is spatially constant, whereas the particle density adjusts locally to this constraint. Thus, equation (5) along the channel leads to Making use of the Maxwell relations implied by equation (4), we finally arrive at This relation allows us to obtain the dependence of the packing fraction on H at constant chemical potential from the normal and lateral pressures ( Supplementary Fig. 7 ). For this purpose, we use the relation , where is the average volume of a particle. How to cite this article: Mandal, S. et al. Multiple reentrant glass transitions in confined hard-sphere glasses. Nat. Commun. 5:4435 doi: 10.1038/ncomms5435 (2014).